Structural bases for the interaction of frataxin with the central components of iron–sulphur cluster assembly Reduced levels of frataxin, an essential protein of as yet unknown function, are responsible for causing the neurodegenerative pathology Friedreich's ataxia. Independent reports have linked frataxin to iron–sulphur cluster assembly through interactions with the two central components of this machinery: desulphurase Nfs1/IscS and the scaffold protein Isu/IscU. In this study, we use a combination of biophysical methods to define the structural bases of the interaction of CyaY (the bacterial orthologue of frataxin) with the IscS/IscU complex. We show that CyaY binds IscS as a monomer in a pocket between the active site and the IscS dimer interface. Recognition does not require iron and occurs through electrostatic interactions of complementary charged residues. Mutations at the complex interface affect the rates of enzymatic cluster formation. CyaY binding strengthens the affinity of the IscS/IscU complex. Our data suggest a new paradigm for understanding the role of frataxin as a regulator of IscS functions. Frataxin is an essential iron-binding protein that is highly conserved in most organisms, from bacteria to humans [1] . Reduced expression levels of this protein are sufficient to induce Friedreich's ataxia, a relentless and currently incurable neurodegenerative disease. Absence of frataxin in knockout mice is also embryonic lethal [2] . Frataxin has been implicated in one of the most important iron-related metabolic pathways through the observation of biochemical and genetic interactions with the highly conserved Nfs1/Isu complex (which corresponds to the IscS and IscU proteins in prokaryotes): Nfs1 and Isu, the two main components central to the iron–sulphur (Fe–S) cluster assembly machinery [3] , [4] , [5] , are, respectively, a cysteine desulphurase enzyme (EC 2.8.1.7), which catalyses the reaction that converts l-cysteine into alanine and a highly reactive sulphide, and the scaffold protein on which the cluster is transiently formed [6] . In addition to having a role in Fe–S cluster assembly, IscS is also involved in other sulphur-related pathways, which include biotin synthesis, tRNA modifications and molybdopterin biosynthesis through interaction with proteins TusA, Thil and MoeB/MoaD [7] , [8] , [9] . Although evidence of a direct interaction between frataxin and the Nfs1/Isu complex has received independent confirmation [3] , [4] , [5] , many questions, the answers to which would be crucial for understanding frataxin function, remain unanswered. For instance, it is unclear as to which of the IscS/IscU components frataxin binds. Calorimetric studies on human frataxin have suggested a direct 1:1 iron-mediated interaction with Isu1 [4] , with nanomolar dissociation constants [10] . In yeast, frataxin (Yfh1) binds to Isu1, but the interaction seems to require Yfh1 oligomerization [11] . In contrast, no direct interaction with isolated IscU was observed for prokaryotic frataxin (CyaY), which interacts instead with IscS [12] , [13] . Another unanswered question is with regard to the role of a highly conserved tryptophan exposed on the frataxin surface [14] , [15] , [16] . Tryptophans are relatively low-occurrence amino acids and their conservation on exposed surfaces strongly suggests a role in molecular recognition [17] . Finally, an even more crucial question is why these interactions take place and, ultimately, what is the primary function of frataxin. This point remains highly controversial. Frataxin has been suggested to function as a chaperone that delivers iron to the IscS/IscU complex [4] , or as a scavenger [18] , which, through formation of large iron-loaded assemblies, prevents iron excesses in mitochondria while still keeping iron biologically available for being delivered to key acceptors. More recently, we have shown that, although not inhibiting desulphurase enzymatic activity, CyaY is able to slow down the speed of Fe–S cluster formation and have proposed a role for frataxin as the gatekeeper of the cluster assembly machinery [13] . Probably the most effective way to test these hypotheses and resolve the debate is to study the frataxin function in vitro , which makes it possible to delimit the system to a minimal and well-controlled number of components. This strategy should allow us to formulate working hypotheses, which could then be tested in vivo . A similar approach has already proven successful, for instance, for the identification of functionally important residues on the frataxin surface [19] . Here, we have dissected the interactions of CyaY, IscS and IscU by gaining information on the structure of their binary and ternary complexes using small-angle X-ray scattering (SAXS), a technique able to provide the overall shape of even large molecular assemblies. We have validated the surfaces of interaction by mapping them directly by nuclear magnetic resonance (NMR) chemical shift perturbation techniques and mutagenesis studies. Finally, we have proven the role of specific residues of either CyaY or IscS on the enzymatic activity of IscS and showed how the presence of CyaY modulates the binding affinities of the complex. As the residues involved in the interaction are conserved, we expect this function to be shared by all frataxin orthologues. The picture suggested by our results is that frataxin is a key element of a complex network of interactions centred on the desulphurase. The interplay between competing interactions may be crucial for regulating cluster formation and selecting alternative metabolic pathways. CyaY forms a 1:1 complex with IscS To quantify the nature of the interaction between Escherichia coli CyaY, IscS and IscU, we measured the stability and stoichiometries of the binary IscS/IscU and IscS/CyaY complexes. We used isothermal calorimetry (ITC), a technique that allows determination of binding constants with high accuracy. Titration of IscS with IscU results in an endothermic binding, which can be fit with a 1:1 binding model and provides a K d of 1.3 ± 0.2 μM ( Fig. 1a ). These results are in agreement with previous data [20] and with the recent structure of the E. coli IscU/IscS complex, which shows interaction of the IscS dimer with two IscU monomers [9] . Titration of IscS with CyaY results in an exothermic reaction, which can also be fit with a 1:1 binding model, leading to a K d of 18.5 ± 2.4 μM ( Fig. 1b ). A lower affinity of IscS for CyaY is in agreement with the evidence that (as opposed to IscU/IscS) the CyaY/IscS complex cannot be easily isolated by gel filtration [21] . As previously described, we could not observe any direct binding between IscU and CyaY either, in the presence of iron, both in aerobic and anaerobic conditions [12] , [13] . 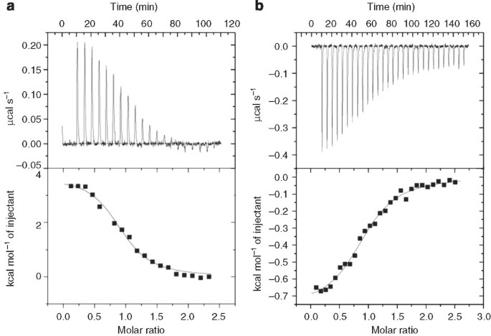Figure 1: Thermodynamic stability of the CyaY/IscS and IscU/IscS complexes. (a) Binding isotherm for the interaction of IscU with IscS. In the upper panel, peaks indicate the heat released after each addition of IscU into the protein solution. In the lower panel, the data were best fit using a single binding constant to calculate the thermodynamic parameters (continuous line). (b) Binding isotherm for the interaction of CyaY with IscS. In the upper panel, peaks indicate the heat released after each addition of CyaY into the protein solution. In the lower panel, the data were fit using a single binding constant. Figure 1: Thermodynamic stability of the CyaY/IscS and IscU/IscS complexes. ( a ) Binding isotherm for the interaction of IscU with IscS. In the upper panel, peaks indicate the heat released after each addition of IscU into the protein solution. In the lower panel, the data were best fit using a single binding constant to calculate the thermodynamic parameters (continuous line). ( b ) Binding isotherm for the interaction of CyaY with IscS. In the upper panel, peaks indicate the heat released after each addition of CyaY into the protein solution. In the lower panel, the data were fit using a single binding constant. Full size image These data provide the first quantification of the affinities of the CyaY/IscS complex and direct evidence that the interaction also occurs without the need of large CyaY assemblies. SAXS reveals the size and shape of the complexes To obtain a molecular description of the IscS/CyaY and IscS/IscU/CyaY complexes, we tried to crystallize the binary complexes. We obtained good-quality crystals under several different conditions, but they invariably contained only IscS [21] . We resorted to a different strategy based on SAXS measurements and molecular modelling validated by experimental data. We acquired and compared SAXS data for each of the isolated individual components, as well as for the binary and ternary complexes (IscS/CyaY, IscS/IscU and IscS/CyaY/IscU). The estimated apparent molecular mass (MM exp ) and hydrated particle volume ( V p ) for IscS agreed with the presence of a dimer in solution ( Fig. 2 and Supplementary Table S1 ), as expected for the constitutive IscS homodimer, which has a P2 symmetry (>90 kDa) [22] . Both IscU and CyaY are monomeric in isolation, in agreement with previous characterizations [23] , [24] , [25] . The MM exp and V p of the complexes are distinctly different from those of the isolated species and correspond to stoichiometries of 1:1:1 for the ternary complex and of 1:1 for both binary complexes. The envelopes of the complexes are clearly different from those of the isolated species, allowing us to identify the excess volumes in which monomeric IscU, CyaY or both could fit ( Fig. 3 ). In agreement with the recently published crystallographic structure, we observed a more elongated shape for the IscS/IscU complex [9] . The shape of the binary complex IscS/CyaY is more globular, thus suggesting that CyaY is located close to the interface between the two IscS protomers. No changes were observed when iron (Fe 2+ ) was aerobically added to the sample to reach a molar ratio of 1:1:2 CyaY/IscS/Fe 2+ (data not shown). 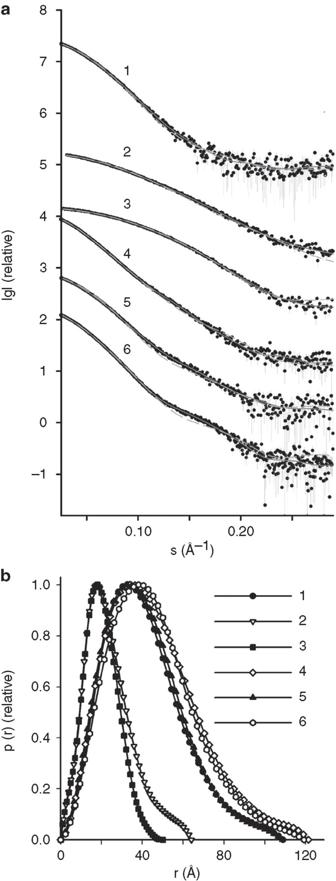Figure 2: Small-angle X-ray scattering data and fits. (a) The X-ray scattering patterns from IscS, IscU, CyaY binary complexes IscS/IscU and IscS/CyaY and ternary complex IscS/CyaY/IscU. The experimental data are displayed as dots with error bars, the scattering from typicalab initiomodels computed by DAMMIF as full lines and the calculated curves from the high-resolution (for proteins alone) and rigid body models (for complexes) computed by CRYSOL/SASREF as dashed lines. Plots display the logarithm of the scattering intensity as a function of momentum transfers=4πsinθ/λ, where 2θis the scattering angle andλis the X-ray wavelength. The successive curves are displayed down by one logarithmic unit for clarity. (b) Distance distribution functions from IscS, IscU, CyaY, binary complexes IscS/IscU and IscS/CyaY and ternary complex IscS/CyaY/IscU (labelled 1–6, respectively). Figure 2: Small-angle X-ray scattering data and fits. ( a ) The X-ray scattering patterns from IscS, IscU, CyaY binary complexes IscS/IscU and IscS/CyaY and ternary complex IscS/CyaY/IscU. The experimental data are displayed as dots with error bars, the scattering from typical ab initio models computed by DAMMIF as full lines and the calculated curves from the high-resolution (for proteins alone) and rigid body models (for complexes) computed by CRYSOL/SASREF as dashed lines. Plots display the logarithm of the scattering intensity as a function of momentum transfer s =4 π sin θ / λ , where 2 θ is the scattering angle and λ is the X-ray wavelength. The successive curves are displayed down by one logarithmic unit for clarity. ( b ) Distance distribution functions from IscS, IscU, CyaY, binary complexes IscS/IscU and IscS/CyaY and ternary complex IscS/CyaY/IscU (labelled 1–6, respectively). 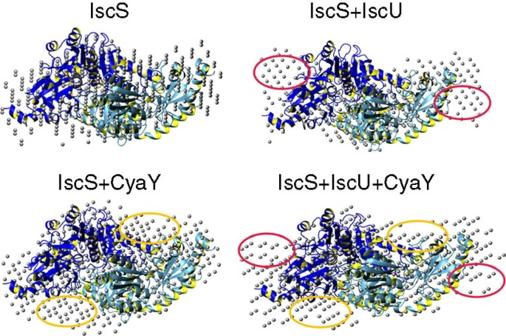Figure 3: Small-angle X-ray scattering shapes. Comparison of the densities superposed to the crystal structures of IscS (1P3W) for IscS alone, IscS/IscU, CyaY/IscS and CyaY/IscS/IscU. Regions with additional density in the binary and ternary complexes are highlighted in red or yellow ovals. Full size image Figure 3: Small-angle X-ray scattering shapes. Comparison of the densities superposed to the crystal structures of IscS (1P3W) for IscS alone, IscS/IscU, CyaY/IscS and CyaY/IscS/IscU. Regions with additional density in the binary and ternary complexes are highlighted in red or yellow ovals. Full size image Multiple runs of the program DAMMIF [26] , a fast version of DAMMIN [27] , were used to produce average low-resolution ab initio shapes for all the constructs. The shape of isolated IscS matches well with the crystal structure (1P3W) [22] ( Fig. 4a ). Among the several NMR and X-ray structures of IscU, the best fit was observed with 1Q48 (ref. 28 ) ( Fig. 4b ), which corresponds to a highly flexible structure in which the N- and C-termini are unfolded. More compact structures such as 2Z7E yielded significantly worse fits ( Fig. 4c ). This is well in agreement with the observation that the N terminus of E. coli IscU is unstructured in solution [21] , [29] . CyaY could be fit with the NMR structure of monomeric CyaY (1SOY) [25] ( Fig. 4d ). 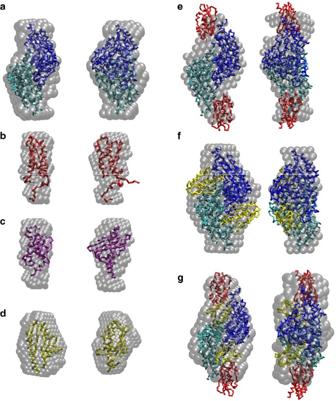Figure 4: Molecular modelling based on small-angle X-ray scattering. Ab initiobead models of IscS (a), the solution (b) and X-ray (c) structures of IscU, CyaY (d), IscU/IscS (e), CyaY/IscS (f) and CyaY/IscS/IscU (g) complexes. The models were obtained from DAMMIF (grey semitransparent spheres) superimposed with rigid body models by the software SASREF. The two components of the crystallographic dimer model of IscS are displayed as cyan and blue Cαtraces. For each model, the right views are rotated counterclockwise around the verticalyaxis. Figure 4: Molecular modelling based on small-angle X-ray scattering. Ab initio bead models of IscS ( a ), the solution ( b ) and X-ray ( c ) structures of IscU, CyaY ( d ), IscU/IscS ( e ), CyaY/IscS ( f ) and CyaY/IscS/IscU ( g ) complexes. The models were obtained from DAMMIF (grey semitransparent spheres) superimposed with rigid body models by the software SASREF. The two components of the crystallographic dimer model of IscS are displayed as cyan and blue C α traces. For each model, the right views are rotated counterclockwise around the vertical y axis. Full size image For all the complexes, rigid body modelling was performed to fit the experimental SAXS data using the high-resolution structures of IscS, IscU and CyaY. The obtained rigid body models displayed good agreement with the ab initio shapes ( Fig. 4e–g ). For the IscS/IscU binary complex, we obtained a better fit with the structure (3LVL) [9] than when using the individual models, thus reinforcing the observation that IscU undergoes a structural transition on binding ( Fig. 4e ). The binary and ternary complexes of CyaY reveal binding of this molecule at a site near the IscS dimer interface, as opposed to IscU, which is positioned towards the periphery of the IscS dimer ( Fig. 4f,g ). Accordingly, the radius of gyration R g and the maximum size of the particle D max for the IscS/IscU complex are significantly larger than for isolated IscS, whereas for IscS/CyaY complex there is only a small increase in these parameters ( Supplementary Table S1 ). The rigid body modelling yielded excellent fits to the scattering data with discrepancies ( χ -values) of <1.45. The fits for the IscS/CyaY and IscS/CyaY/IscU models displayed minor deviations at higher angles (beyond s -values of 0.15 Å −1 ). These deviations can be explained by the presence of small populations of free components in solution, in agreement with the lower affinity of the IscS/CyaY complex as compared with the IscS/IscU one (the difference is of approximately one order of magnitude). Overall, the ab initio and rigid body models from SAXS are consistent with each other and give us the first direct picture of the structure of the IscS/IscU/CyaY complexes. Model validation and collection of further restraints To validate the SAXS models and obtain more restraints for further modelling, we resorted to NMR techniques that, by detecting spectral perturbation, are a sensitive tool to identify even residual binding and map the information to specific residues. We used 2 H, 15 N double-labelled CyaY and titrated it with IscS up to a 1:1 molar ratio. Perdeuteration was found to be necessary to decrease spin diffusion, resulting in much sharper spectra and therefore in a higher resolution. The residues of CyaY most affected by addition of IscS are Trp14, Leu15, Glu19, Asp22, Asp23, Trp24, Asp25, Asp27, Ser28, Asp29, Ile30, Asp31, Cys32, Glu33, Ile34, Leu39, Thr42, Phe43, Glu44 and Gly46 ( Fig. 5a ). These residues map spatially close in the region of CyaY comprising α1, β1 and the α1β1 loop (blue side chains in Fig. 5b ). We then added IscU to the solution up to a 1:1:1 molar ratio (CyaY/IscS/IscU) and observed new spectral perturbations ( Fig. 5c ). Some of the residues already perturbed by IscS, that is, 14, 19, 22–24, 27–31, 33–34, 39 and 43–44, were further affected by the addition of IscU. In addition, other residues, namely, Thr40, Ile41, Lys48, Ile50, Asp52, Arg53, Glu55, Trp61, Leu62, Ala63, Thr64, Gln66, Gly68, Tyr69 and His70, were either shifted and/or broadened. They mostly map to the β-sheet surface (red side chains in Fig. 4b ). In particular, both the backbone and the indole amides of Trp61 were affected. The additional perturbation must be caused either by a direct contact of these residues with IscU or by a conformational change induced by the addition of this component. 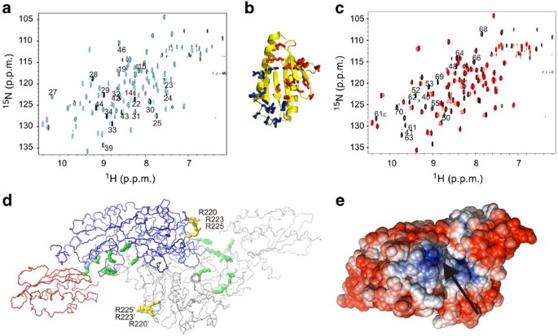Figure 5: Experimental validation of the models. (a) Superposition of the hetero single quantum coherence spectra of15N uniformly labelled CyaY (light blue) with the final point of a titration with unlabelled IscS (1:1 molar ratio, black). (b) Residues of CyaY (1SOY) involved in the interaction with IscS (blue) and IscU (red). (c) Superposition of the hetero single quantum coherence spectra of the CyaY/IscS complex (black) with the final point of titration with unlabelled IscU (up to 1:1:1 molar ratios, red). (d) Mapping of IscS mutations into the IscS/IscU crystal structure (3LVL). To highlight the symmetry relation, the backbone of one of the IscS protomers is shown in blue with the complexed IscU shown in red, whereas the backbones of the corresponding symmetry related to IscS/IscU are shown in grey. A linear fog effect was applied. The side chains of mutated residues, which have no effect on the interaction with CyaY, are shown in green, those that abolish interaction are shown in yellow. The dimer interface and the presence of IscU delimit a small cavity in which CyaY is accommodated. (e) Electrostatic surface of unbound IscS. An arrow indicates the position of the positively charged patch involved in binding. The patch comprises residues arginines 55, 67, 219–220, 223, 225 and 237. The residues 220, 223 and 225 are those that, if mutated to glutamates, abolish CyaY binding. IscS is oriented as indand rotated by 90° around the horizontalxaxis. Figure 5: Experimental validation of the models. ( a ) Superposition of the hetero single quantum coherence spectra of 15 N uniformly labelled CyaY (light blue) with the final point of a titration with unlabelled IscS (1:1 molar ratio, black). ( b ) Residues of CyaY (1SOY) involved in the interaction with IscS (blue) and IscU (red). ( c ) Superposition of the hetero single quantum coherence spectra of the CyaY/IscS complex (black) with the final point of titration with unlabelled IscU (up to 1:1:1 molar ratios, red). ( d ) Mapping of IscS mutations into the IscS/IscU crystal structure (3LVL). To highlight the symmetry relation, the backbone of one of the IscS protomers is shown in blue with the complexed IscU shown in red, whereas the backbones of the corresponding symmetry related to IscS/IscU are shown in grey. A linear fog effect was applied. The side chains of mutated residues, which have no effect on the interaction with CyaY, are shown in green, those that abolish interaction are shown in yellow. The dimer interface and the presence of IscU delimit a small cavity in which CyaY is accommodated. ( e ) Electrostatic surface of unbound IscS. An arrow indicates the position of the positively charged patch involved in binding. The patch comprises residues arginines 55, 67, 219–220, 223, 225 and 237. The residues 220, 223 and 225 are those that, if mutated to glutamates, abolish CyaY binding. IscS is oriented as in d and rotated by 90° around the horizontal x axis. Full size image Validation of the surface of interaction on IscS, as suggested by SAXS, came from the design of IscS mutants, chosen to target residues that could potentially affect interaction with CyaY ( Fig. 5d ). A IscS_R220E/R223E/R225E triple mutant was designed to invert the charge of a positively charged patch formed by residues 55, 67, 219–220, 223, 225 and 237 (all arginines) close to the dimer interface ( Fig. 5e ). These mutations affect solvent exposed residues. Therefore they do not alter the stability of the protein but are expected to abolish binding to the complementary charged surface of CyaY. IscS_I314E/M315E, IscS_K101E/K105E, IscS_E334S/R340S and IscS_R39E/W45E mutants were also produced as controls. Because affecting residues far from the CyaY/IscS interface, these mutations introduce charge inversion and/or perturb the surface but leave invariant the interaction. The effects of these mutants on the NMR spectrum of CyaY were tested and compared with that of wild-type IscS. The only mutant that caused no perturbation of the CyaY spectrum is IscS_R220E/R223E/R225E (data not shown), thus indicating that these mutations are sufficient to abolish the interaction completely. The other mutants produced the same perturbation as the CyaY spectrum, as observed for wild-type IscS. Following the same strategy, the mutants were tested for IscU binding as well, and yielded results fully consistent with the structure of the IscS/IscU complex [9] , thus providing an independent validation of our procedure ( Supplementary Discussion ). Taken together, these results lend further support to the SAXS models, positioning CyaY in a site well distinct from that occupied by IscU. The interaction between IscU and CyaY is mediated by IscS A hybrid approach combining SAXS-based rigid body modelling (SASREF [30] ) with the docking software HADDOCK [31] was used to build the refined models of the complexes. Whereas the nominal resolution of the SAXS-based models is defined by the maximum momentum transfer in the fitting range of Figure 2 (2 π / s max ∼ 10–20Å), the use of experimental docking restraints and high-resolution structures in hybrid modelling is expected to significantly push the resolution limit for the consensus model, thus allowing for meaningful analysis of protein–protein interactions in the complex. The consensus model reflects most of the experimental observables and suggests several novel observations. Although occupying distinct surfaces of IscS, CyaY and IscU are next to each other, with CyaY fitting the cavity delimited by the IscS dimer interface and the IscU-binding site ( Fig. 6a ). This region overlaps only partially with that occupied by TusA, another protein partner of IscS involved in delivering sulphur for tRNA modification [7] ( Fig. 6b ). Compared with the position of TusA [9] , CyaY is inserted less deeply into the cleft formed by IscU and the IscS dimer interface, as directly supported by the fact that IscS_R39E_W45E retains binding to CyaY, whereas these two residues were shown to be directly involved in the interaction with TusA ( Supplementary Table S2 ). On the other hand, mutation of R220 and the surrounding positively charged residues of IscS abolishes CyaY but not TusA binding. 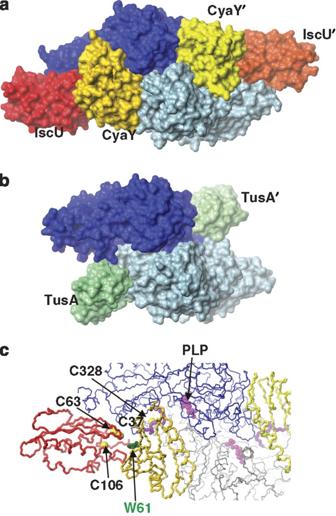Figure 6: Structure of the ternary complex CyaY/IscS/IscU. (a) Surface representation of the model obtained by combining the small-angle X-ray scattering and NMR information, showing in blue and cyan the two IscS protomers; in red and orange red, IscU; and in gold and yellow, CyaY. (b) Surface representation in the same orientation as in (a) of the IscS complex (blue and light blue) with TusA9(different gradations of green, 3LVJ). (c) Blowup of Figure 6a but in a ribbon representation showing the relative position of pyridoxal phophate (PLP, magenta), the catalytic loop (purple), the three conserved cysteines of IscU (yellow) and Trp61 of CyaY (green). The catalytic loop was built by homology using the 3GZC47 coordinates the sequence of which has a sequence similarity/identity of 30 and 50%, respectively, and superposes to 1P3W, with a lower root mean square deviation of 1.21 Å. The resulting model was energy minimized by the Gromacs package55. Figure 6: Structure of the ternary complex CyaY/IscS/IscU. ( a ) Surface representation of the model obtained by combining the small-angle X-ray scattering and NMR information, showing in blue and cyan the two IscS protomers; in red and orange red, IscU; and in gold and yellow, CyaY. ( b ) Surface representation in the same orientation as in ( a ) of the IscS complex (blue and light blue) with TusA [9] (different gradations of green, 3LVJ). ( c ) Blowup of Figure 6a but in a ribbon representation showing the relative position of pyridoxal phophate (PLP, magenta), the catalytic loop (purple), the three conserved cysteines of IscU (yellow) and Trp61 of CyaY (green). The catalytic loop was built by homology using the 3GZC47 coordinates the sequence of which has a sequence similarity/identity of 30 and 50%, respectively, and superposes to 1P3W, with a lower root mean square deviation of 1.21 Å. The resulting model was energy minimized by the Gromacs package [55] . Full size image CyaY sits relatively close to the loop containing the catalytic Cys328, but far from the pyridoxal phophate ( ~ 18 Å), in agreement with our previous observation that CyaY does not interfere with enzymatic activity [13] ( Fig. 6c ). Conversely, although we do not know its exact position, as it is not visible in the crystal structures, the catalytic loop is, in principle, long enough to protrude and contact the nearby CyaY. The experimental restraints that position the region 18–36 of CyaY to pack against the region of IscS containing Arg220, Arg223 and Arg225 automatically also impose the surface of the β-sheet of CyaY to be spatially close to IscU. Although insufficient to stabilize a stand-alone CyaY/IscU complex, the surface of interaction between these two proteins may stabilize the ternary complex. Among the residues of CyaY that are spatially proximal to IscU is the exposed Trp61, which is close to, albeit not necessarily in contact with, the conserved cysteines of IscU. CyaY influences the kinetics of enzymatic Fe–S cluster assembly We have previously shown that the presence of CyaY slows down the enzymatic rates of Fe–S cluster formation, suggesting a role of frataxin as an IscS inhibitor [13] . To investigate whether the interaction of CyaY with the IscS/IscU complex has a direct influence on these inhibitory properties, we tested the effect of replacing wild-type IscS with its mutants on the rates of cluster formation. We followed this process by analysing, under strict anaerobic conditions, the absorption spectrum at 456 nm, a wavelength typical of the cluster [20] . For comparison, we also tested two CyaY mutants, CyaY_E18K/E19K/E22 K and CyaY_W61R. The first should affect the surface of interaction with IscS and therefore have complementary effects to those of IscS_R220E/R223E/R225E. The second should influence the surface of interaction with IscU. The presence of CyaY has a strong inhibitory effect as compared with the assay carried out in its absence, and appreciably reduces the initial reaction rate ( Fig. 7a , a red curve as compared with a green curve). The IscS_R220E/R223E/R225E and CyaY_E18K/E19K/E22K mutants behave as the control experiment in the absence of CyaY (blue and magenta curves), as expected from abolishing the interaction between CyaY and the enzyme. CyaY_W61R has an intermediate behaviour, suggesting that this mutation causes a lower degree of disruption of the complex. IscS_I314E/M315E, which weakens without abolishing the interaction between IscS and IscU, only results in a reduction of the kinetic rates (cyan curve). The other IscS mutants that should have no effect on the complex behave similar to the wild-type IscS (data not shown). 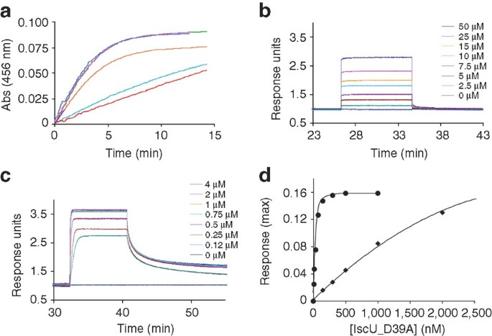Figure 7: Influence of complex formation on the kinetics of cluster formation and on the complex affinities. (a) Kinetics rates of Fe–S cluster formation on IscU. The experiments are all conducted under the same conditions (1 μM IscS or IscS mutants, 25 μM Fe2+, 50 μM IscU, 250 μM Cys, 2 mM DTT and 5 μM of CyaY or CyaY mutants). Green curve: control experiment in the absence of CyaY; red curve: control experiment in the presence of wild-type CyaY; blue, magenta, orange and cyan curves: experiments carried out by substituting wild-type proteins with CyaY_E18K_E19K_E22K, IscS_R220E_R223E_R225E, CyaY_W61R and IscS_I314E_M315E, respectively. (b) Biolayer interferometry profile of the titration of CyaY with increasing concentrations of IscS in the absence of IscU. (c) As in b, but in the presence of IscU. Because the complex is stabilized, lower concentrations of IscS are needed to reach saturation. (d) Plot of the interferometry response obtained by immobilizing IscS as a function of increasing concentrations of cluster-free (circle) and cluster-loaded (diamond) IscU_D39A mutant. Figure 7: Influence of complex formation on the kinetics of cluster formation and on the complex affinities. ( a ) Kinetics rates of Fe–S cluster formation on IscU. The experiments are all conducted under the same conditions (1 μM IscS or IscS mutants, 25 μM Fe 2+ , 50 μM IscU, 250 μM Cys, 2 mM DTT and 5 μM of CyaY or CyaY mutants). Green curve: control experiment in the absence of CyaY; red curve: control experiment in the presence of wild-type CyaY; blue, magenta, orange and cyan curves: experiments carried out by substituting wild-type proteins with CyaY_E18K_E19K_E22K, IscS_R220E_R223E_R225E, CyaY_W61R and IscS_I314E_M315E, respectively. ( b ) Biolayer interferometry profile of the titration of CyaY with increasing concentrations of IscS in the absence of IscU. ( c ) As in b, but in the presence of IscU. Because the complex is stabilized, lower concentrations of IscS are needed to reach saturation. ( d ) Plot of the interferometry response obtained by immobilizing IscS as a function of increasing concentrations of cluster-free (circle) and cluster-loaded (diamond) IscU_D39A mutant. Full size image Taken together, these results provide a strong and convincing link between the interaction of the three components and the enzyme activity. CyaY enhances the affinity of IscU on IscS Finally, we wondered whether binding of one component on IscS has an influence on the affinities of the other interactions and whether the presence of the cluster on IscU could decrease the affinity of the IscU/IscS complex, thus suggesting how Fe–S cluster formation could be regulated. We measured the dissociation constants by Biolayer interferometry (BLI), a novel technique that measures molecular interactions and also provides information on the on/off rates. When we immobilized CyaY on the surface and measured the affinities of the CyaY/IscS complex in the absence of IscU, we obtained a K d of 23±3 μM ( Fig. 7b ), whereas when IscU was present, the K d is 35±6 nM ( Fig. 7c ). Vice versa, by immobilizing IscS on the surface, the affinitiy value of the IscU/IscS interaction in the absence of CyaY is 1.5±0.3 μM. When the experiment was repeated in the presence of CyaY, we measured a K d of 400±30 nM, which is appreciably lower than the value observed in the binary complex. In all cases, we observed that the dissociation rates ( k off ) of the ternary complex were lower than those observed for the binary complexes (for example, the k off for the disassembly of the IscS/IscU complex is 0.8 s −1 in the absence of CyaY, versus 0.006 s −1 in the presence of CyaY). The values obtained by BLI are in excellent agreement with ITC results, which also provide a K d for the IscU/IscS interaction in the presence of CyaY that is approximately one order of magnitude tighter than that observed in the absence of CyaY (250±18 nM data not shown). We then tried to measure the affinities of the IscU/IscS interaction for cluster-free and cluster-loaded IscU (in the absence of CyaY) to check whether the presence of the cluster is able to modulate the interaction with IscS. Unfortunately, the cluster is too unstable when bound to wild-type IscU, especially under non-anaerobic conditions, to allow us to perform interferometry assays. We thus used an IscU_D39A mutant that is known to stabilize the cluster that persists for several hours, even under aerobic conditions [32] , [33] . We measured by BLI a K d of 41.7±4 nM for the cluster-free IscU mutant. The presence of CyaY further increases the affinity yielding to a K d of 12.00±2 nm. Conversely, we obtained a K d of 0.86±0.04 μM for the cluster-loaded protein ( Fig. 7d ). Taken together, these results indicate that the presence of the third component and/or the iron state of IscU modulate the affinities of the binary IscU/IscS and CyaY/IscS complexes. We have reported a description of the structural determinants of the interaction between bacterial frataxin and IscS and IscU, the two essential components of isc operon. We have shown that IscS binds CyaY with a 1:1 stoichiometry that reflects the twofold symmetry of the dimeric enzyme. We then resorted to SAXS to obtain a more detailed, although low-resolution, description of the complexes. The information was validated by NMR and by judiciously designed mutations and finally translated into a comprehensive three-dimensional model. These results help us to address several open questions. As the interaction with IscS occurs at the level of CyaY monomers, there is no need for the large assemblies that have been suggested to be involved in the recognition of yeast frataxin (Yfh1) by the corresponding Nfs1/Isu1 complex [11] . The surfaces of interaction that we have mapped both on desulphurase and CyaY are anyway incompatible with the binding of a large assembly: CyaY is accommodated in a relatively narrow cavity of the IscS dimer, which could not accommodate larger species without a major rearrangement. Even more important is the consideration that the residues involved in the Yfh1 trimer interfaces (the trimer being the smallest building block for larger spherical assemblies) are the same that mediate IscS recognition [34] . Our findings also resolve the long-standing debate on whether frataxin interacts with IscS and/or with IscU. A direct interaction between human frataxin and Isu was reported as early as 2003 [4] . These results could not, however, be reproduced in pulldowns of the bacterial orthologues, either using overexpressed proteins or endogenous extracts [12] , [13] , suggesting the possibility that IscU could be detected solely as a consequence of its interaction with IscS. Direct titrations of the two proteins using biophysical techniques also failed to detect an interaction [13] , [21] . We now show that CyaY packs mainly against IscS, which functions as a mould. Contacts with IscU are possible but only in the context of the ternary complex. However, it is possible that the differences observed between prokaryotic and eukaryotic proteins may be explained by the N-terminal extension present only in eukaryotic frataxins. These additional residues, which are a flexible spacer between the mitochondrial localization signal and frataxin, could contribute to stabilizing the interaction with Isu, thus explaining why this can be observed in the absence of desulphurase only in eukaryotes. Interestingly, IscU recognition seems to involve CyaY Trp61, as directly suggested by the SAXS models and the NMR data. This interaction could explain the high degree of conservation of the Trp throughout the frataxin family and the severe effects that mutation of this residue have in vitro and in vivo [35] , [36] . Even though we should not at this stage overspeculate, as the resolution we are working at is insufficient to discuss atomic details, it is clear from our data that formation of the IscS/IscU/CyaY complex does not require the presence of iron. This is at variance with previous reports. Pulldown experiments on the yeast complex have suggested iron to be essential for the interaction [3] . In another study, it was suggested that binding of Yfh1 requires oligomerization and occurs in an iron-independent manner [11] . However, the surface of interaction involves a direct recognition of the negatively charged region of CyaY by a positively charged patch on IscS, thus rendering an active role of iron in complex formation unlikely. We confirmed our previous observation that CyaY slows down Fe–S cluster formation and proved that the effect is directly related to the interaction between CyaY and IscS [13] . This behaviour could be explained in several ways. First, CyaY could directly affect the enzymatic properties of IscS. However, the catalytic site is in a region close but quite distinct from those hosting IscU and CyaY in our structure, in full agreement with our previous findings that conversion of cysteine into alanine is unperturbed by the presence of CyaY [13] . Second, CyaY could interfere with the cluster transfer from IscS to IscU, for instance, by impairing the motions of the flexible catalytic loop containing Cys328. Evidence that nucleotide modification, which is one of the alternative functions of IscS, is not impaired by CyaY-overproducing conditions, seems, however, to also disprove this possibility [9] . A different explanation is directly suggested by our data. We observe that formation of the ternary complex increases the affinities of the interaction between IscU (and of IscU_D39A) and IscS and decreases the dissociation rate constants. The inhibitory effect of CyaY on the enzymatic kinetics could then be the consequence of an impairment of the detachment of IscU from IscS, because of the stabilizing effect of CyaY. This hypothesis implies that, once the cluster is formed, cluster-loaded IscU detaches from IscS to transfer the cluster to the next acceptor and regenerate the reaction, a possibility that is reasonable because the surface of IscU that hosts the cluster is buried in the complex [9] . Accordingly, we have observed an appreciably different affinity of the cluster-free and cluster-loaded forms at least of the IscU_D39A mutant. IscU is also known to interact with the chaperone HscA, another component of the isc operon required for Fe–S cluster assembly or delivery from IscU to target proteins, with a site at least partially overlapping with the surface involved in IscS recognition [37] . Taken together, these observations suggest the following cycle, even though still awaiting a much deeper description of the exact time sequence of the events. CyaY and IscU are likely to be simultaneously bound to IscS, thus stabilizing the complex and allowing cluster formation. Once the cluster is loaded on IscU, this would detach from IscS, having a reduced affinity (as hinted by our results with the IscU_D39A mutant) and the interaction being competed out by the chaperone HscA. The complex IscU/HscA, further stabilized by the cochaperone HscB [38] , [39] , would deliver the cluster to the final acceptors. Once freed from the cluster, IscU and CyaY would bind to IscS again, thus restarting the cycle. Other competitors might interfere with CyaY and further regulate the process. What does all this tell us about the cellular function of frataxin? It is increasingly clear that the role of frataxin cannot simply be that of an iron chaperone, as it would be hard to understand in such a case why frataxin binds the IscU/IscS complex with the same surface that transports iron or why its presence affects the complex stability and the kinetics of Fe–S cluster formation. We suggest a role for frataxin as the regulator of a complex network, centred on the desulphurase of multiple and competing interactions, the nature of which we are just starting to understand. IscS is known to bind not only IscU and CyaY but also the small component of the isc operon YfhJ (also known as IscX) [40] , [41] and various other proteins involved in completely different pathways, such as TusA, Thil and MoeB/MoaD [6] , [7] , [9] . With the only exception of MoeB/MoaD, which is still undetermined, these interactions have all been mapped in distinct but partially overlapping surfaces of IscS [9] . The different affinities of these proteins for IscS may determine which of these partners will be bound at any one time. The iron-loaded state of at least some of the proteins (for example, iron loaded/iron free, cluster loaded/cluster free) and the relative cellular concentrations may add additional opportunities for achieving regulation. In conclusion, although much more work is needed to completely clarify the cellular role of frataxin, establishment of the structural bases of its interaction with IscS/IscU opens a new perspective to further advance the field. The information provided in this work may be crucial for understanding both, one of the most essential metabolic pathways and the molecular basis of Friedreich's ataxia. Protein purification E. coli CyaY, IscS, IscU and IscU_D39A mutants were purified as previously described [14] , [21] , [23] . In short, they were produced as fusion proteins with a His-tagged glutathione-S-transferase and purified by affinity chromatography using Ni-NTA agarose gel (Qiagen). The cells overexpressing IscU were grown in Luria broth-enriched medium containing 8.3 μM ZnSO 4 to stabilize the protein fold [21] , [28] , [29] . All purification steps were carried out in the presence of 20 mM β-mercaptoethanol. The collected proteins were cleaved overnight from glutathion-S-transferase by Tobacco Etch Virus protease and further purified by gel-filtration chromatography on a Superdex 75 26/60 column (GE Healthcare). Protein purity was checked by SDS–polyacrylamide gel electrophoresis and by mass spectrometry. SAXS measurements and modelling SAXS data were collected on the EMBL X33 beamline on the storage ring DORIS III (DESY) [42] . IscS, CyaY and IscU solutions and their complexes were measured at 15 °C in a concentration range of 2.5–5.0 mg ml −1 . As CyaY binds both Fe(II) and Fe(III), ferrous ammonium sulphate was added to reach a 1:1:2 CyaY/IscS/Fe molar ratio under aerobic conditions. The data were recorded using a 1 M PILATUS detector (DECTRIS) at a sample-detector distance of 2.7 m and a wavelength of 1.5 Å, covering the range of momentum transfer 0.012< s <0.6 Å −1 . No measurable radiation damage was detected by comparison of four successive time frames with 30 s exposures. The data were averaged after normalization to the intensity of the transmitted beam and the scattering of the buffer was subtracted using PRIMUS [42] . Forward scattering I (0) and the radius of gyration R g were evaluated using the Guinier approximation [43] . These parameters were also computed from the entire scattering patterns using the program GNOM [44] , which provides the distance distribution functions p ( r ) and the maximum particle dimensions D max . The solute MM exp was estimated by comparison of the forward scattering with that from reference solutions of bovine serum albumin (MM 66 kDa). The excluded volume of the hydrated particle (the Porod volume V p ) was computed as reported by Porod [45] . Low-resolution ab initio models of IscS, IscU, CyaY and their complexes were generated by the program DAMMIF [26] , which represents the protein by an assembly of densely packed beads. Simulated annealing was used to build a compact interconnected configuration of beads that fits the experimental data I ( s ) to minimize discrepancy: where N is the number of experimental points, c is a scaling factor, I calc ( s j ) and σ ( s j ) are the calculated intensity and the experimental error at the momentum transfer s j , respectively [27] . The results from 10 separate runs were averaged to determine common structural features using the program DAMAVER [46] . The models were further refined by rigid body modelling using the program SASREF [30] which uses an simulated annealing protocol to generate an interconnected assembly of subunits without steric clashes that fits the scattering data. The coordinates 1P3W and 1SOY were assumed for isolated IscS and CyaY [22] , [25] . As the loop containing Cys328 is not visible in the 1P3W, this was built by homology from the 3GZC [47] structure and energy minimized. Several structures of IscU were tested. The coordinates of the 1Q48 entry [28] were finally selected as those giving the best fit to the data and the best overlap to the ab initio envelope of isolated IscU. The scattering amplitudes of the individual subunit structures were calculated using the program CRYSOL [48] . Docking was performed with a combination of SASREF [30] and HADDOCK 1.3 (ref. 31 ) software, using 3LWL and 1SOY as the starting structures. To improve the resolution, we incorporated the following information. We assumed P2 symmetry for the complexes. Arginines 220, 223 and 225 of IscS were imposed to interact with residues 22–48 of CyaY on the basis of mutagenesis and NMR titrations. For testing purposes, modelling was also achieved without these restraints and provided similar quality fits and similar positions of IscU/CyaY relative to the IscS structure. The accuracy of the resulting models was validated by considering not only our own results (mutagenesis and NMR studies) but also literature data [9] ( Supplementary Table S2 ). Solutions that did not fulfil all the mutagenesis data were discarded. NMR titrations NMR spectra were acquired on 15 N uniformly labelled CyaY or IscU samples and 15 N- 2 H- 13 C uniformly labelled CyaY samples in 90%/10% H 2 O/D 2 O. All proteins used in the titration experiments, both labelled and non-labelled, were in 20 mM HCl-Tris at pH 8.0, in 150 mM NaCl and in 20 mM β-mercaptoethanol. All spectra were recorded at 25 °C on a Varian spectrometer operating at 800 MHz 1 H frequencies or on a Bruker spectrometer operating at 700 MHz 1 H frequencies and equipped with 5 mm triple-resonance probes or cryoprobes. Water suppression was achieved by the WATERGATE sequence [49] . The spectra were processed with NMRPipe [50] and analysed with XEASY [51] . ITC measurements Complex formation between IscU and IscS was measured by ITC using a MicroCal VP-ITC microcalorimeter (MicroCal) [52] . Proteins were dialysed overnight into the same buffer (20 mM Tris–HCl at pH 8.0, 150 mM NaCl and 10 mM β-mercaptoethanol). When anaerobic conditions were necessary (that is, for testing the CyaY/IscU interaction in the presence of Fe 2+ ), the solutions were thoroughly degassed and prepared in an anaerobic chamber(Belle technology). The experiments were conducted at 25 °C. The sample cell typically contained IscS (16–25 μM or 180–200 μM concentrations) and the syringe contained either IscU (180–250 μM) or CyaY (1.7–1.9 mM). For the studies of the IscS/IscU/CyaY ternary complex, the sample cell contained IscS (16–25 μM) saturated by CyaY (380–420 μM). Heat of dilution, as determined by titrating IscU or CyaY into the buffer alone and subtracted from the raw titration data before analysis, was always negligible as compared with the heat signal observed for the initial titrant additions. Data were fit by least-squares procedures using Microcal Origin (version 7.0) provided by the manufacturer. All titrations using IscU were fit using the 'ligand in the cell' assumption. K d values were averaged over three measurements. Biolayer interferometry All experiments were conducted aerobically in 20 mM HEPES pH 7.5, 150 mM NaCl, 2 mM tris(2-carboxyethyl)phosphine and 0.5 mg ml −1 bovine serum albumin on an Octet Red instrument (ForteBio), operating at 25 °C. Streptavidin-coated biosensors with immobilized biotinylated IscS were exposed to different concentrations of IscU (0–5 μM) in the presence and absence of 100 μM CyaY or to cluster-free and cluster-loaded IscU_D39A mutant (0–4 μM). Alternatively, streptavidin-coated biosensors with immobilized biotinylated CyaY were exposed to different concentrations of IscS (0–50 μM) in the presence and absence of 10 μM IscU. Fe–S cluster reconstitution on IscU or IscU_D39A Cluster reconstitution was performed under strict anaerobic conditions in a chamber (Belle technology) kept under nitrogen atmosphere. The reaction was followed by absorbance spectroscopy using a Cary 50 Bio spectrophotometer (Varian). Variations in the absorbance at 456 nm were measured as a function of time. A solution of 50 μM IscU was incubated in sealed cuvettes typically using 3 mM DTT and 25 μM Fe(NH 4 ) 2 SO 4 for 30 min in 50 mM Tris–HCl buffer, pH 7.5 and 150 mM NaCl. The reaction was initiated by adding IscS (1 μM) and the reaction substrate cysteine (250 μM). The relative concentrations of the assay components were chosen as previously detailed [8] . In short, the concentration of IscU, which is the final cluster acceptor in the assay, was set to 50 μM, that is, a value that allowed us to easily measure the ultraviolet signal of the cluster. IscS was set to catalytic concentrations (1 μM) to avoid even minimal contributions of unspecific iron-thiolate polysulphides bound to IscS [53] . The IscS/IscU molar ratio also determines the time scale in which the kinetics are completed [54] . Similarly, we used small concentrations of CyaY (typically 5 μM). The presence of the antioxidant DTT is necessary to provide reducing equivalents required for cluster generation and to regenerate the prosthetic group pyridoxal phophate [20] . Fe–S cluster reconstitution on the IscU_D39A mutant was obtained using the same protocol as for wild-type IscU and incubating the protein in anaerobic conditions for 4 h at room temperature. How to cite this article: Prischi, F. et al . Structural bases for the interaction of frataxin with the central components of iron–sulphur cluster assembly. Nat. Commun. 1:95 doi: 10.1038/ncomms1097 (2010).